Regulation ofFTsplicing by an endogenous cue in temperate grasses Appropriate flowering timing is crucial for plant reproductive success. The florigen, FLOWERING LOCUS T (FT), interacts with 14-3-3 proteins and the bZIP transcription factor FD, functioning at core nodes in multiple flowering pathways. There are two FT homologues, FT1 and FT2, in Brachypodium distachyon . Here we show that FT2 undergoes age-dependent alternative splicing (AS), resulting in two splice variants ( FT2α and FT2β ). The FT2β -encoded protein cannot interact with FD or 14-3-3s but is able to form heterodimers with FT2α and FT1, thereby interfering with the florigen-mediated assembly of the flowering initiation complex. Notably, transgenic plants overproducing FT2β exhibit delayed flowering, while transgenic plants in which FT2β is silenced by an artificial microRNA display accelerated flowering, demonstrating a dominant-negative role of FT2β in flowering induction. Furthermore, we show that the AS splicing of FT2 is conserved in important cereal crops, such as barley and wheat. Collectively, these findings reveal a novel posttranscriptional mode of FT regulation in temperate grasses. The correct timing of the transition from the vegetative to the reproductive stage is a critical point during plant life cycles. Plants require appropriate environmental conditions, including optimal photoperiod and temperature, to stimulate flowering at a specific time of the year. Additionally, plants also must develop to a certain age with fixed amounts of hormones to achieve flowering [1] . As the encoder of the mobile flower-promoting signal florigen, the FLOWERING LOCUS T ( FT ) gene has been shown to have key roles in integrating external and endogenous cues to control the onset of flowering. FT proteins are a clade of the phosphatidylethanolamine-binding protein (PEBP) family, which act as highly conserved regulators in plants that relay signals from upstream to downstream in flowering pathways. In Arabidopsis thaliana , FT messenger RNA (mRNA) gradually increases with developmental time under a long-day (LD) photoperiod [2] . After synthesis in leaves, FT protein travels through the vasculature to the shoot apical meristem (SAM) and interacts with a bZIP transcription factor, named FD, which is expressed specifically in the SAM [3] , [4] . Subsequently, the FT/FD complex activates a number of MADS box genes, including APETALA1 , FRUITFULL and SUPPRESSOR OF OVEREXPRESSION OF CONSTANS 1 to stimulate floral organ initiation [5] . The 14-3-3 proteins, a family of regulatory molecules conserved in animal and plants, can directly interact with the FT homologue Heading date 3a in rice apical shoots, forming a functional complex that translocates to the nucleus [6] . Thus, 14-3-3 proteins may function as scaffold proteins to associate FT with FD to trigger flowering. Numerous FT transcriptional regulators have been identified to date. For example, in A. thaliana , CONSTANS and GIGANTEA activate FT expression in the photoperiod pathway [7] , [8] , [9] , while FLOWERING LOCUS C and SHORT VEGETATIVE PHASE form a MADS-box complex that negatively mediates FT expression in the flowering vernalization-related pathway [10] . Two well-known plant-conserved microRNAs (miRNAs), miR156 and miR172, directly or indirectly act at the FT region through their targets, mediating age-dependent flowering processes [11] , [12] , [13] . Compared with the extensive knowledge of FT control at the transcriptional level, our understanding of FT regulation at the posttranscriptional level is limited. Temperate grasses, including wheat and barley, are major sources of food and biofuel worldwide. Some specialized components, lacking orthologues in A. thaliana and rice, have been discovered in temperate grasses and can affect FT gene expression in day-length and vernalization flowering pathways [14] , [15] , [16] . The typical Pooideae grass Brachypodium distachyon has been considered as a suitable model system for investigating gene function in temperate cereals because of its small genome, simple growth requirements and short life cycle [17] . Phytochrome C, rather than phytochrome A or B, is an essential light receptor for photoperiodic flowering in wheat and B. distachyon , suggesting that there are different evolutionary features of LD flowering responses in temperate grasses [18] , [19] , [20] . Moreover, a Pooideae -specific miRNA, miR5200, has recently been identified that directly silences two FT orthologues and has a crucial role in the photoperiod-mediated flowering pathway in B. distachyon , further implying that a distinct flowering control mechanism exists in temperate cereals [14] . Alternative splicing (AS) is a universal mechanism that produces multiple mRNAs from one gene through the variable selection of splice sites during mRNA generation [21] , [22] . AS can modulate gene expression levels by introducing a premature termination codon, resulting in the degradation of a special RNA-splicing isoform through a nonsense-mediated decay pathway [23] . Additionally, different transcript isoforms may produce truncated proteins that may have different subcellular localization, stability level or function [23] . Several studies have implicated the involvement of AS in plant development, circadian rhythm, starch metabolism, hormone signaling and abiotic stress response, as well as pathogen defense [24] , [25] , [26] , [27] , [28] , [29] , [30] , [31] , [32] , [33] , [34] , [35] , [36] , suggesting that this mechanism of gene regulation has a significant role in plant adaptation and evolution. Despite the revelation by next-generation sequencing that AS occurs in >60% of A. thaliana and 42% of B. distachyon genes, the biological significance of most AS events in plants is still largely unknown [21] , [37] , [38] , [39] . Previously, we demonstrated that two orthologous FT genes, FTL1 ( Bradi2g07070 ) and FTL2 ( Bradi1g48830 ), have miR5200-targeting sites and are regulated by miR5200 in B. distachyon [14] . Because in B. distachyon , more amino acids of FTL2, compared with FTL1, are identical with those of florigen VRN3 in wheat and barley, we re-designated FTL1 as FT2 and FTL2 as FT1 to be clearer when analyzing the phylogenetic relationships among the FTs of temperate grasses [40] . In this study, we show that AS of FT2 has an important role in controlling florigen activity by producing a competitive repressor in B. distachyon . FT2 β, which only lacks a short section of the N-terminal PEBP domain, can attenuate the activities of the flowering initiation complex by interacting with full-size FT2α and FT1. The FT2 β/ FT2α ratio progressively decreased with plant growth, resulting in a slow gradual increase in the florigen activity level. The overexpression of FT2β in transgenic plants resulted in delayed flowering, whereas plants with downregulated FT2β activity through artificial miRNA-induced repression, exhibited accelerated flowering, further demonstrating that FT2 β acts as a dominant-negative repressor in flowering time control in B. distachyon . Together, these results reveal a novel molecular mode of FT posttranscriptional regulation in temperate grasses. FT2 is subject to AS generating two isoforms In B. distachyon , FT1 and FT2 share high amino-acid sequence identity and their overproduction gives rise to extremely early bolting phenotypes, indicating that they perform redundant roles in flowering initiation [14] , [15] , [40] . During the study of the regulatory mechanism of FT1 and FT2 in flowering, we interestingly found that two PCR products were generated by a pair of FT2 primers, implying the existence of FT2 AS in B. distachyon ( Fig. 1a ). By comparing the two FT2 cDNA sequences, we discovered that one splicing product was missing 84 nucleotides at the 5′-end of the first exon compared with a typical FT gene.Thus we designated this form as FT2β and the full-size transcript as FT2α ( Fig. 1b ). A protein sequence alignment showed that the missing 28 amino acids came from the 5′ terminal region of the PEBP domain of FT2β, which is more variable compared with the middle and 3′ regions ( Fig. 1c ; Supplementary Fig. 1a ). However, no FT1 splicing variant was detected in B. distachyon , possibly because the gene structure of FT1 is different from that of FT2 ( Supplementary Fig. 1b,c ). 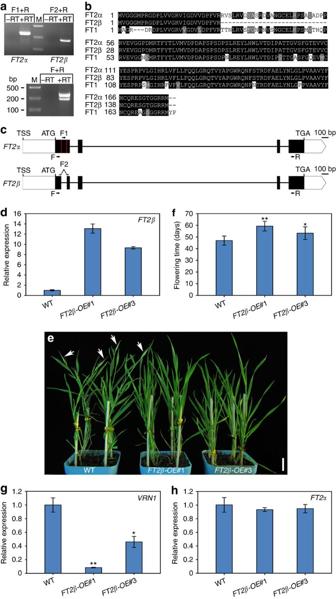Figure 1: Identification ofFT2AS inB. distachyon. (a) Detection of alternatively splicedFT2transcripts by RT-PCR. F1 and F2 are specific forward primers forFT2αandFT2βamplification, respectively, while primer F is used forFT2αandFT2βPCR simultaneously. R is the reverse primer. RT, reverse transcription. M, marker. bp, base pairs. (b) Protein sequence alignment of different FT2 alternative isoforms and FT1. (c) Schematic genomic structure ofFT2splicing variants. White boxes indicate untranslated regions and black boxes indicate exons. TSS indicates the transcriptional start site. (d) qRT-PCR analysis ofFT2βexpression in wild-type Bd21 and the indicatedFT2β-OEtransgenic plants. Three four-week-oldB. distachyonplants were pooled and collected for RNA isolation.UBC18was used as an internal control for normalization of qRT-PCR results. qRT-PCR analyses were performed in three biological replicates with similar results. The point represents the mean value of three technical replicates in a representative biological experiment. Error bars indicate s.d. (e) Representative phenotype ofFT2βoverexpressing transgenic plants.White arrows point to spikes. Scale bar, 2 cm. (f) Flowering time of wild-type and the indicatedFT2β-OEtransgenic plants. Error bars indicate s.d. (n=13). Student’st-test, **P<0.01, *P<0.05. (g) qRT-PCR analysis of downstream flowering geneVRN1expression in wild-type and the indicatedFT2β-OEtransgenic plants. The four-week-old whole plant tissues including leaves and shoot apex were collected forVRN1examination. qRT-PCR analyses were performed in three biological replicates with similar results. The point represents the mean value of three technical replicates in a representative biological experiment. Error bars indicate s.d. Student’st-test, **P<0.01, *P<0.05. (h) qRT-PCR analysis ofFT2αexpression levels in wild-type and the indicatedFT2β-OEtransgenic plants. Figure 1: Identification of FT2 AS in B. distachyon . ( a ) Detection of alternatively spliced FT2 transcripts by RT-PCR. F1 and F2 are specific forward primers for FT2α and FT2β amplification, respectively, while primer F is used for FT2α and FT2β PCR simultaneously. R is the reverse primer. RT, reverse transcription. M, marker. bp, base pairs. ( b ) Protein sequence alignment of different FT2 alternative isoforms and FT1. ( c ) Schematic genomic structure of FT2 splicing variants. White boxes indicate untranslated regions and black boxes indicate exons. TSS indicates the transcriptional start site. ( d ) qRT-PCR analysis of FT2β expression in wild-type Bd21 and the indicated FT2β-OE transgenic plants. Three four-week-old B. distachyon plants were pooled and collected for RNA isolation. UBC18 was used as an internal control for normalization of qRT-PCR results. qRT-PCR analyses were performed in three biological replicates with similar results. The point represents the mean value of three technical replicates in a representative biological experiment. Error bars indicate s.d. ( e ) Representative phenotype of FT2β overexpressing transgenic plants.White arrows point to spikes. Scale bar, 2 cm. ( f ) Flowering time of wild-type and the indicated FT2β-OE transgenic plants. Error bars indicate s.d. ( n =13). Student’s t -test, ** P <0.01, * P <0.05. ( g ) qRT-PCR analysis of downstream flowering gene VRN1 expression in wild-type and the indicated FT2β-OE transgenic plants. The four-week-old whole plant tissues including leaves and shoot apex were collected for VRN1 examination. qRT-PCR analyses were performed in three biological replicates with similar results. The point represents the mean value of three technical replicates in a representative biological experiment. Error bars indicate s.d. Student’s t -test, ** P <0.01, * P <0.05. ( h ) qRT-PCR analysis of FT2α expression levels in wild-type and the indicated FT2β-OE transgenic plants. Full size image Using specific primers to amplify each FT2 RNA splicing product, we detected the presence of both variants in B. distachyon in most cases ( Fig. 1a ). Most AS events in plants are shown to be affected by ambient temperature fluctuations [24] , [25] , [28] , [41] . Similarly, the ratios of FT2β/FT2α were altered when plants were grown at high temperatures ( Supplementary Figs 2 and 3 ). To determine the role, if any, of different FT2 variants in the control of flowering, we attempted to independently overproduce FT2α and FT2β in B. distachyon . As previously described by us and others, the ectopic expression of intact FT2 ( FT2α ) in B. distachyon leads to very early flowering and arrested vegetative growth [14] , [40] , demonstrating the positive florigen activity of FT2α. Next, we generated FT2β overexpression ( FT2β-OE ) transgenic plants and determined the flowering time in their T 1 generations under LD conditions. Wild-type and transgenic plants displayed similar rates of vegetative development. However, eight independent positive FT2β-OE plants exhibited significantly late heading dates compared with wild-type and the null segregants of the transgenic plants ( Supplementary Fig. 4 ). Because FT2β-OE#1 and FT2β-OE#3 displayed a severe and mild delay of flowering time, respectively, we chose their T 3 homozygous plants for further molecular and phenotypic analyses. Quantitative real-time PCR (qRT-PCR) showed that FT2β was approximately 12- and 9-fold higher in FT2β-OE#1 and FT2β-OE#3 plants, respectively, than in the parental wild-type ( Fig. 1d ; Supplementary Fig. 5a,b ). FT2β-OE#1 bolted 12 days (59 versus 47 days) and FT2β-OE#3 bolted more than 6 days (53 versus 47 days) later than wild-type plants under LD conditions ( Fig. 1e,f ). Furthermore, the expression of VRN1 , an APETALA1 orthologue acting downstream of FT in temperate grasses, was dramatically reduced in FT2β-OE#1 and FT2β-OE#3 plants ( Fig. 1g ; Supplementary Fig. 5c,d ). The FT2β-OE plants exhibited wild-type levels of FT2α mRNA, excluding the possibility that the late flowering of FT2β-OE was caused by the suppression of FT2α expression ( Fig. 1h ; Supplementary Fig. 5e,f ). Thus FT2α and FT2β may have different effects on floral transition in B. distachyon. FT2β does not interact with FD or 14-3-3 proteins In A. thaliana and rice, during transport from leaves to SAM, florigen interacts with several 14-3-3 proteins in the cytoplasm and subsequently translocates to the nucleus to bind FD and form a flowering activation complex. The interaction of TaFDL2, the FD-like protein in wheat, with FT1 and FT2 has been previously demonstrated [4] , [42] .Thus we cloned its orthologue from B. distachyon and assigned the same name as in wheat ( Supplementary Fig. 6 ). To address whether FT2α and FT2β in B. distachyon can form a flowering initiation complex with FD, we first used yeast two-hybrid assays to determine their interactions with FDL2. Strong interactions were detected between FT2α and FDL2 in yeast cells. However, there was no detectable binding of FT2β to FDL2 in yeast ( Fig. 2a ). To verify these results, we examined the associations between the two FT2 isoforms and FDL2 using bimolecular fluorescence complementation (BiFC) assays with a split yellow fluorescent protein (YFP) system in Nicotiana benthamiana leaf mesophyll cells. As shown in Fig. 2b , there was a strong fluorescent signal in the nucleus when FT2α was transiently co-expressed with FDL2. By contrast, no YFP fluorescence could be detected in leaves co-expressing FT2β and FDL2, suggesting that FT2β cannot bind FDL2 in vivo . Co-immunoprecipitation (Co-IP) assays further confirmed a strong binding between FT2α and FDL2 but no interaction between FT2β and FDL2 ( Fig. 2c ). 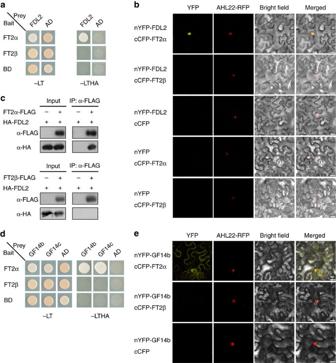Figure 2: Interaction analysis of FT2α and FT2β with FD-like and 14-3-3 proteins. (a) Interaction analysis of FT2α and FT2β with FD-like protein (FDL2) in yeast cells. Yeast cell growth on selective media without Leu, Trp, His and Ade (−LTHA) indicates positive interactions. (b) BiFC interaction assays of FT2α and FT2β with FDL2. Partial YFP fusion constructs were expressed transiently inN. benthamianaleaves. AHL22-RFP was used as a nuclear marker. Scale bar, 20 μm. (c)In vivoCo-IP assays of two FT2 splicing isoforms with FDL2. FLAG-tag FT2α or FLAG-tag FT2β were co-expressed with HA-tag FDL2 inN. benthamianaleaves. (d) Yeast two-hybrid analyses of interactions between FT2 isoforms and two 14-3-3 proteins (GF14b and GF14c). (e) BiFC interaction assays of FT2α and FT2β with 14-3-3 protein GF14b. Scale bar, 20 μm. Figure 2: Interaction analysis of FT2α and FT2β with FD-like and 14-3-3 proteins. ( a ) Interaction analysis of FT2α and FT2β with FD-like protein (FDL2) in yeast cells. Yeast cell growth on selective media without Leu, Trp, His and Ade (−LTHA) indicates positive interactions. ( b ) BiFC interaction assays of FT2α and FT2β with FDL2. Partial YFP fusion constructs were expressed transiently in N. benthamiana leaves. AHL22-RFP was used as a nuclear marker. Scale bar, 20 μm. ( c ) In vivo Co-IP assays of two FT2 splicing isoforms with FDL2. FLAG-tag FT2α or FLAG-tag FT2β were co-expressed with HA-tag FDL2 in N. benthamiana leaves. ( d ) Yeast two-hybrid analyses of interactions between FT2 isoforms and two 14-3-3 proteins (GF14b and GF14c). ( e ) BiFC interaction assays of FT2α and FT2β with 14-3-3 protein GF14b. Scale bar, 20 μm. Full size image Similar to Heading date 3a in rice, wheat FT1 can also interact with two 14-3-3 proteins, GF14b and GF14c [6] , [42] .Thus we selected several B. distachyon 14-3-3 proteins including GF14b and GF14c to determine their abilities to interact with FT2α and FT2β ( Fig. 2d ; Supplementary Fig. 7a ). Both GF14b and GF14c interacted with FT2α in the yeast two-hybrid and BiFC assays ( Fig. 2d,e ). In contrast, FT2β did not bind to any 14-3-3 proteins ( Fig. 2d,e ; Supplementary Fig. 7b ). Thus 14-3-3 proteins may not form bridges with FT2β to trigger flowering in B. distachyon . Together, these observations suggest that FT2 splicing variants may have different actions, with one forming a flowering activation complex as a result of direct physical interactions with 14-3-3s and FD, while the other has lost this ability. FT2β attenuates the bindings of florigen to FD and 14-3-3s Genetic engineering experiments have shown that unnatural splicing variants can act as dominant-negative mutants to interrupt the activities of wild-type isoforms [24] , [25] , [28] . FT2β’s inability to bind to FD and 14-3-3s implied that it may interfere with flowering activation complex formation. To test this possibility, we expressed FT2β in yeast cells, which contained BD-FT2α and AD-FDL2 fusions ( Fig. 3a ). β-Galactosidase (β-Gal) activity assays revealed that the expression of FT2β substantially repressed FT2α-FD binding ( Fig. 3b ). Likewise, the interaction between FT2α and GF14b in yeast three-hybrid systems was significantly reduced when FT2β was expressed ( Fig. 3b ). 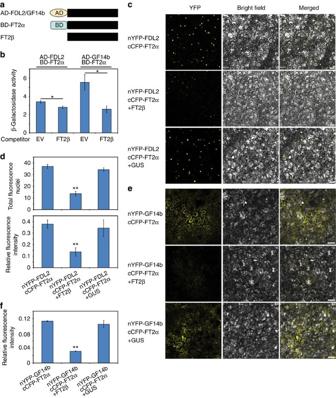Figure 3: Attenuation of FT2α-binding capacity with FD-like and 14-3-3 proteins by FT2β. (a) Constructs used for yeast three-hybrid assays. FT2β was used as the competitor to the interacting proteins with activation domain (AD) and DNA-binding domain (BD). (b) Relative quantification of inhibition activities of FT2β in yeast three-hybrid assays. β-Gal activities were measured in the presence or absence of FT2β (Student’st-test, *P<0.05). Bars indicate s.e.m. of three replicates. EV, empty vector. (c) Representative photographs of fluorescence signals in BiFC assays for determination of FT2β effects on FT2α and FDL2 interactions inN. benthamianaleaf cells. GUS was used as a control in the absence of FT2β. Scale bar, 50 μm. (d) Total fluorescence nuclei and relative fluorescence intensity in BiFC assays used for analyses of FT2β inhibition activities to FT2α and FDL2 interactions. Bars indicate s.e.m. of three replicates (Student’st-test, **P<0.01). (e) Representative photographs showing the fluorescence signals in BiFC assays for determination of FT2β effects on FT2α and 14-3-3 interactions inN. benthamianaleaf cells. GUS was used as a control in the absence of FT2β. Scale bar, 50 μm. (f) Relative fluorescence intensity in BiFC assays used for determination of FT2β-inhibitory activities to FT2α and 14-3-3 interactions. Bars indicate s.e.m. of three replicates (Student’st-test, **P<0.01). Figure 3: Attenuation of FT2α-binding capacity with FD-like and 14-3-3 proteins by FT2β. ( a ) Constructs used for yeast three-hybrid assays. FT2β was used as the competitor to the interacting proteins with activation domain (AD) and DNA-binding domain (BD). ( b ) Relative quantification of inhibition activities of FT2β in yeast three-hybrid assays. β-Gal activities were measured in the presence or absence of FT2β (Student’s t -test, * P <0.05). Bars indicate s.e.m. of three replicates. EV, empty vector. ( c ) Representative photographs of fluorescence signals in BiFC assays for determination of FT2β effects on FT2α and FDL2 interactions in N. benthamiana leaf cells. GUS was used as a control in the absence of FT2β. Scale bar, 50 μm. ( d ) Total fluorescence nuclei and relative fluorescence intensity in BiFC assays used for analyses of FT2β inhibition activities to FT2α and FDL2 interactions. Bars indicate s.e.m. of three replicates (Student’s t -test, ** P <0.01). ( e ) Representative photographs showing the fluorescence signals in BiFC assays for determination of FT2β effects on FT2α and 14-3-3 interactions in N. benthamiana leaf cells. GUS was used as a control in the absence of FT2β. Scale bar, 50 μm. ( f ) Relative fluorescence intensity in BiFC assays used for determination of FT2β-inhibitory activities to FT2α and 14-3-3 interactions. Bars indicate s.e.m. of three replicates (Student’s t -test, ** P <0.01). Full size image To further investigate the negative effects of FT2β on flowering activation complex formation, we transiently co-expressed FT2β with split YFP-tagged FT2α and FDL2 proteins in N. benthamiana leaf mesophyll cells. Compared with the GUS protein, which was expressed instead of FT2β as a control, the numbers of fluorescent cell nuclei, as well as the intensity of fluorescence, generated by the interaction of FT2α and FDL2 was reduced when FT2β was co-expressed ( Fig. 3c,d ). Meanwhile, in line with the yeast three-hybrid assay results, competition BiFC experiments also showed a repressive effect of FT2β on the association of FT2α with GF14b in the cytoplasm of N. benthamiana leaf cells ( Fig. 3e,f ). Because FT1 and FT2 may have redundant roles in flowering initiation [4] , [14] , [40] , we investigated whether FT2β could affect the efficiency of flowering induction complex formed by FT1, in addition to that formed by FT2α. Indeed, FT2β had an inhibitory effect in the competition BiFC assay ( Supplementary Fig. 8 ). Collectively, these results indicate that FT2β functions as a repressor of the formation of the flowering initiation complex containing FT1, FT2α, 14-3-3s and FD. FT2β forms heterodimers with FT2α and FT1 FT2β suppresses the interactions of florigen proteins with FD and 14-3-3s; however, we did not detect any physical interactions of FT2β with FDL2 or 14-3-3s ( Fig. 2 ). Thus we next investigated another possible mechanism. It has been suggested that heterodimers may be generated by different splicing isoforms [24] , [25] , [28] , thus we investigated whether FT2β was able to form a heterodimer with FT2α to produce a nonfunctional protein complex. To test this possibility, we first performed a yeast two-hybrid analysis and observed a strong interaction between FT2α and FT2β ( Fig. 4a ). The formation of a heterodimer between FT2α and FT2β was also detected in the nuclei as well as in the cytoplasm of N. benthamiana leaf cells using BiFC assays ( Fig. 4b ). Furthermore, a yeast two-hybrid analysis showed an interaction of FT2β with FT1, suggesting that FT2β is able to form heterodimers with both florigen proteins ( Supplementary Fig. 9 ). 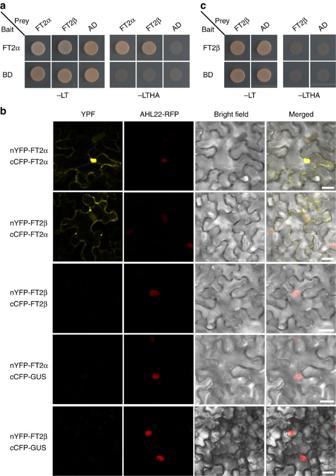Figure 4: Homodimer and heterodimer formation analyses between FT2α and FT2β. (a) FT2α can form homodimer and heterodimer with FT2β in yeast cells. (b) BiFC assays for FT2α and FT2β homodimer and heterodimer formation determination. GUS was used as a control in the absence of FT2α or FT2β. Scale bar, 20 μm. (c) FT2β cannot form homodimer in yeast cells. Yeast cell growth on selective media without Leu, Trp, His and Ade (−LTHA) indicates positive interactions. Figure 4: Homodimer and heterodimer formation analyses between FT2α and FT2β. ( a ) FT2α can form homodimer and heterodimer with FT2β in yeast cells. ( b ) BiFC assays for FT2α and FT2β homodimer and heterodimer formation determination. GUS was used as a control in the absence of FT2α or FT2β. Scale bar, 20 μm. ( c ) FT2β cannot form homodimer in yeast cells. Yeast cell growth on selective media without Leu, Trp, His and Ade (−LTHA) indicates positive interactions. Full size image Interestingly, yeast two-hybrid and BiFC assays revealed that both FT2α and FT1, but not FT2β, could form homodimers ( Fig. 4a–c ; Supplementary Fig. 9 ). Thus we propose that the negative effect of FT2β on flowering time results from the binding of FT2β to FT2α and FT1, which prevents them from interacting with FD and 14-3-3s, thereby reducing the number of functional flowering initiation complexes. FT2 AS is controlled by an endogenous cue Having discovered a molecular mode by which FT2β represses flowering, we wondered when FT2β contributes to the regulation of floral initiation in B. distachyon . Unlike in A. thaliana , temperature has a very limited impact on the timing of phase transition from the vegetative to reproductive stage in B. distachyon [43] ; therefore, FT2 splicing may have little, if any, relevance to temperature-mediated flowering, even though the FT2β / FT2α ratio can change in response to the environmental temperature. Previously, we reported that FT1 and FT2 transcription level gradually increase with development under LD conditions in B. distachyon [14] . Thus we asked whether FT2 AS changes with plant age. Using a qRT-PCR analysis with splicing-variant-specific amplification primers, the ratio of FT2β / FT2α abundance was found to decline during plant growth ( Fig. 5a,b ; Supplementary Figs 10 and 11 ). Although the transcription levels of FT2α and FT2β gradually increased throughout plant development as a result of photoperiodic induction, the proportions of different FT2 -splicing isoforms changed with increasing plant age. FT2β accumulated to a much higher level than FT2α during the first 4 weeks, but FT2α rose much faster than FT2β afterwards ( Fig. 5a ; Supplementary Figs 10 and 11 ), thereby resulting in a gradual decrease in the FT2β / FT2α ratio as development progressed ( Fig. 5b ). 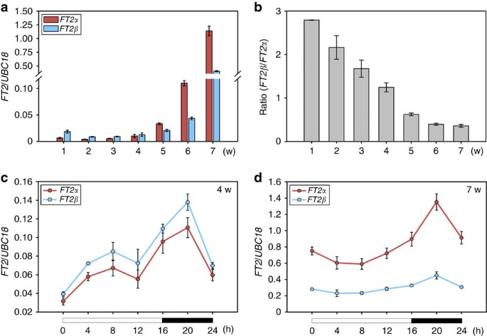Figure 5: Age-dependentFT2AS. (a) Expression analysis ofFT2αandFT2βalong with different age. Upper flat leaves from five Bd21 plants with the indicated age were pooled and collected for RNA isolation. Each qRT-PCR analysis was performed in three biological replicates with similar results. The point represents the mean value of three technical replicates in a representative biological experiment. The transition from vegetative to reproductive stage of Bd21 plants occurs at 4–5 weeks. Standard curve forFT2α,FT2βandUBC18quantification is shown inSupplementary Fig. 2. The absolute value ofFT2α,FT2βandUBC18is shown inSupplementary Fig. 10a. Error bars indicate s.d. w, weeks. (b)FT2β/FT2αratio during plant development. (c) and (d) Diurnal expression analysis ofFT2αandFT2βin 24-h period when plants were 4 and 7 weeks old. The absolute value ofFT2α,FT2βandUBC18at each time point is shown inSupplementary Fig. 12. Upper flat leaves from five Bd21 plants at the indicated time were pooled and collected for RNA isolation. The white and black bars along the horizontal axes represent light and dark periods, respectively. The numbers below the horizontal axes indicate the time in hours. Error bars indicate s.d. h, hours, w, weeks. Figure 5: Age-dependent FT2 AS. ( a ) Expression analysis of FT2α and FT2β along with different age. Upper flat leaves from five Bd21 plants with the indicated age were pooled and collected for RNA isolation. Each qRT-PCR analysis was performed in three biological replicates with similar results. The point represents the mean value of three technical replicates in a representative biological experiment. The transition from vegetative to reproductive stage of Bd21 plants occurs at 4–5 weeks. Standard curve for FT2α , FT2β and UBC18 quantification is shown in Supplementary Fig. 2 . The absolute value of FT2α , FT2β and UBC18 is shown in Supplementary Fig. 10a . Error bars indicate s.d. w, weeks. ( b ) FT2β/FT2α ratio during plant development. ( c ) and ( d ) Diurnal expression analysis of FT2α and FT2β in 24-h period when plants were 4 and 7 weeks old. The absolute value of FT2α , FT2β and UBC18 at each time point is shown in Supplementary Fig. 12 . Upper flat leaves from five Bd21 plants at the indicated time were pooled and collected for RNA isolation. The white and black bars along the horizontal axes represent light and dark periods, respectively. The numbers below the horizontal axes indicate the time in hours. Error bars indicate s.d. h, hours, w, weeks. Full size image To further determine the effects of increasing age on FT2 AS, we examined the diurnal expression rhythms of FT2α and FT2β in 4- and 7-week-old B. distachyon leaves. As shown in Fig. 5c and Supplementary Fig. 12 , the FT2β expression level was higher than that of FT2α in 4-week-old plants during the day–night cycle. By contrast, more FT2α accumulated than FT2β in 7-week-old plants ( Fig. 5d ; Supplementary Fig. 12 ), further confirming the development-dependent change in FT2 AS. Therefore, in addition to the transcriptional control of FT , the posttranscriptional regulation of FT by AS may also contribute to flowering at the appropriate time in B. distachyon . We propose that a high level of FT2β in young plants may prevent precocious flowering, which allows plants to accumulate sufficient biomass to produce enough seeds to propagate the next generation. Down regulation of FT2β induces early flowering We previously found that the overexpression of miR5200, which simultaneously targets both FT1 and FT2 , led to a severe delay of flowering onset in B. distachyon [14] , suggesting that the suppression of FT2α expression may result in late flowering. To further characterize the role of FT2β in flowering control, we attempted to use artificial miRNAs to knock down FT2β expression, because artificial miRNA can specifically silence one splicing variant but not the other. In plants, most of miRNAs start with a 5′uridine (U) for their correct sorting into ARGONAUTE 1 (AGO1) silencing complex [44] . However, there is no adenine (A) nucleotide available for the design of artificial miRNA with a 5′U across the FT2β transcripts that skips the exon nucleotides of FT2α ( Supplementary Fig. 13a ). Even beginning with a 5′A, miR172 can be properly loaded into AGO1-silencing effectors as a result of its specific secondary structure [44] . Thus we designed an artificial miRNA using MIR172a as a backbone to downregulate FT2β ( Fig. 6a ; Supplementary Fig. 13a,b ). We successfully obtained eight independent transgenic Bd21-3 plants and termed them amiRFT2β . RNA analysis revealed high accumulation of artificial miRNA and are resultant decrease of FT2β expression in typical transgenic plants ( Fig. 6b,c ; Supplementary Fig. 14a,b ). In addition,we did not find reductions in the gene expression levels of FT2α or other potential amiRFT2β targets in amiRFT2β plants ( Fig. 6d ; Supplementary Figs 14c,d and 15 ), suggesting that our artificial miRNA, which was introduced into plants, can specifically act on the desired transcripts. 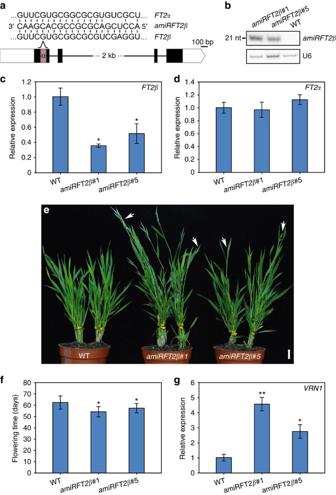Figure 6: Interruption of FT2β activity by artificial miRNA results in early flowering. (a) Schematic diagram ofamiRFT2β. (b) Northern blotting analysis of artificial miRNA accumulation inamiRFT2βtransgenic plants. U6 was used as a loading control for RNA gel blot. (c) qRT-PCR analysis ofFT2βexpression in wild-type Bd21-3 and the indicatedamiRFT2βtransgenic plants.UBC18was used as an internal control for normalization of qRT-PCR results. Three six-week-oldB. distachyonplants were pooled and collected for RNA isolation. Each qRT-PCR analysis were performed in three biological replicates with similar results. The point represents the mean value of three technical replicates in a representative biological experiment. Error bars indicate s.d. Student’st-test, *P<0.05 (d) qRT-PCR analysis ofFT2αexpression in wild-type and the indicatedamiRFT2βtransgenic plants. (e) Representative photograph of flowering phenotypes inamiRFT2βtransgenic and wild-type Bd21-3 plants. White arrows point to spikes. Scale bar, 2 cm. (f) Flowering time of wild-type and the indicated two lines ofamiRFT2βtransgenic plants. Error bars indicate s.d. (n=10). Student’st-test, *P<0.05 (g) qRT-PCR analysis of flowering downstream geneVRN1expression in wild-type and the indicatedamiRFT2βtransgenic plants. Total RNA from 5-week-old whole-plant tissues, including leaves and shoot apex, were used forVRN1examination. Student’st-test, **P<0.01, *P<0.05. Figure 6: Interruption of FT2β activity by artificial miRNA results in early flowering. ( a ) Schematic diagram of amiRFT2β . ( b ) Northern blotting analysis of artificial miRNA accumulation in amiRFT2β transgenic plants. U6 was used as a loading control for RNA gel blot. ( c ) qRT-PCR analysis of FT2β expression in wild-type Bd21-3 and the indicated amiRFT2β transgenic plants. UBC18 was used as an internal control for normalization of qRT-PCR results. Three six-week-old B. distachyon plants were pooled and collected for RNA isolation. Each qRT-PCR analysis were performed in three biological replicates with similar results. The point represents the mean value of three technical replicates in a representative biological experiment. Error bars indicate s.d. Student’s t -test, * P <0.05 ( d ) qRT-PCR analysis of FT2α expression in wild-type and the indicated amiRFT2β transgenic plants. ( e ) Representative photograph of flowering phenotypes in amiRFT2β transgenic and wild-type Bd21-3 plants. White arrows point to spikes. Scale bar, 2 cm. ( f ) Flowering time of wild-type and the indicated two lines of amiRFT2β transgenic plants. Error bars indicate s.d. ( n =10). Student’s t -test, * P <0.05 ( g ) qRT-PCR analysis of flowering downstream gene VRN1 expression in wild-type and the indicated amiRFT2β transgenic plants. Total RNA from 5-week-old whole-plant tissues, including leaves and shoot apex, were used for VRN1 examination. Student’s t -test, ** P <0.01, * P <0.05. Full size image An analysis of the flowering time of these transgenic plants, in the T 3 generation, under LD conditions revealed early heading ( Fig. 6e ). The heading date was earlier by an average of 8 days in amiRFT2β compared with those of control plants (54 versus 62 days, on average) ( Fig. 6f ). Consistent with these phenotypic observations, VRN1 expression was two fold to four fold higher in amiRFT2β than in wild-type plants ( Fig. 6g ; Supplementary Fig. 14e,f ). The extent of early flowering phenotype in different amiRFT2β lines correlated with the mature artificial miRNA accumulation as well as the reduced FT2β expression, suggesting that the acceleration of flowering by reduced FT2β activity is likely due to the formation of more flowering activation complex and the resulting enhanced VRN1 expression. To help exclude the possibility that the early flowering in amiRFT2β is due to the unspecific effects of the artificial miRNA, we generated amiRFT2α transgenic lines, which specifically silenced FT2α expression by introducing a different artificial miRNA that targeted the intron region of FT2α where it is different from that of FT2β ( Supplementary Fig. 13 ). We observed a severe delay of flowering (94 versus 68 days) and a reduction in VRN1 expression in strong amiRFT2α lines ( Supplementary Figs 16 and 17 ). Weak amiRFT2α lines exhibited comparable heading dates with those of wild-type plants ( Supplementary Figs 16 and 17 ). This may be because of the limited decrease in FT2α expression or the redundant activities of FT1 and FT2 in B. distachyon . The lack of early flowering phenotypes in all four amiRFT2α lines suggested that the precocious heading of amiRFT2β was due to the compromised FT2β activity rather than the unspecific effects of the artificial miRNA. Taken together, the acceleration and delay in heading dates in amiRFT2β and a miRFT2α plants, respectively, further indicated that FT2β and FT2α have antagonistic roles in the flowering processes of B. distachyon . Dynamic change in FT2 AS is prevalent in temperate grasses In light of the opposite roles of FT2 splicing isoforms in B. distachyon flowering control demonstrated above, we asked whether the age-dependent modulation of FT2 AS was conserved among other plants. Using RT-PCR, similar splicing variants of FT2 orthologues in A. thaliana , rice and maize were not detected, even though the gene structures of the FT2 homologous genes in rice and maize are the same as that in B. distachyon ( Supplementary Fig. 18 ). As B. distachyon belongs to Pooideae , we investigated whether AS of FT2 is present in other temperate grasses. Indeed, we found two splicing variants of FT2 in Aegilops tauschii , wheat and barley, which differed by the loss of nucleotides that encode the same amino acids as in B. distachyon ( Supplementary Fig. 19 ). Additionally, we observed that wheat and barley FT2β were expressed at much lower levels than FT2α in 8-week-old plants, whereas FT2α transcripts were less abundant in 2-week-old plants ( Fig. 7a,b ). These results suggest that the change in the AS of FT2 regulated by development is conserved in temperate grasses. 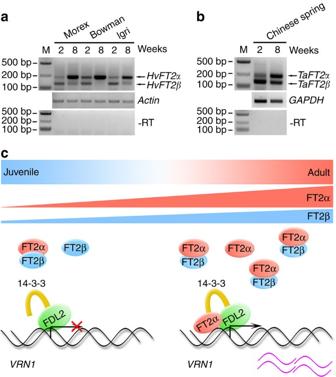Figure 7: Dynamic changesinFT2AS with plant development is prevalent in barley and wheat. (a) RT-PCR analysis ofFT2αandFT2βexpression in barley with the indicated age. Primers designed for simultaneous amplification ofFT2αandFT2βin a single PCR reaction were used. Total RNA from three typical varieties of barley was isolated for reverse transcription. M, marker. (b) RT-PCR analysis ofFT2αandFT2βexpression in wheat with different ages. Total RNA from Chinese Spring was isolated for reverse transcription. (c) A working model for two FT2 splicing isoforms during plant flowering-induction processes in temperate grasses. Although both twoFT2splicing transcripts increase along with plant development, their increasing rates are not consistent, resulting in distinctFT2β/FT2αratio with different age. FT2β and FT2α can form heterodimers. Thus when plants are vegetative, the formation of flowering-induction complex is blocked, becauseFT2βexpression level is higher than that ofFT2α. When plants grow to reproductive stage, more FT2α accumulates than FT2β, and the flowering initiation complex can be formed in the SAM to induceVRN1expression, ensuring eventual plant flowering at right growth phase. Figure 7: Dynamic changesin FT2 AS with plant development is prevalent in barley and wheat. ( a ) RT-PCR analysis of FT2α and FT2β expression in barley with the indicated age. Primers designed for simultaneous amplification of FT2α and FT2β in a single PCR reaction were used. Total RNA from three typical varieties of barley was isolated for reverse transcription. M, marker. ( b ) RT-PCR analysis of FT2α and FT2β expression in wheat with different ages. Total RNA from Chinese Spring was isolated for reverse transcription. ( c ) A working model for two FT2 splicing isoforms during plant flowering-induction processes in temperate grasses. Although both two FT2 splicing transcripts increase along with plant development, their increasing rates are not consistent, resulting in distinct FT2β / FT2α ratio with different age. FT2β and FT2α can form heterodimers. Thus when plants are vegetative, the formation of flowering-induction complex is blocked, because FT2β expression level is higher than that of FT2α . When plants grow to reproductive stage, more FT2α accumulates than FT2β, and the flowering initiation complex can be formed in the SAM to induce VRN1 expression, ensuring eventual plant flowering at right growth phase. Full size image AS is a common gene regulatory mechanism that greatly increases the complexity of transcripts and proteins encoded by an organism’s genome. From high-throughput transcriptome studies in plants, it is now clear that AS is much more prevalent than previously estimated [37] . However, when, how and why these splicing variants are generated remains, to a large extent, unknown [22] , [23] . In this study, we reported that the highly conserved flowering integrator gene, FT , is also subjected to AS in temperate grasses. FT2β can heterodimerize with FT2α and FT1 in plant leaves and is unable to bind FD and 14-3-3s at the shoot apex, resulting in its interference with the formation of flowering inductive complexes. Thus it has a dominant-negative role in controlling flowering onset. The importance of change in FT2 AS during development was demonstrated by the alteration in heading date timing, which results from artificial-miRNA induced reduction in FT2β activity in B. distachyon ( Fig. 6 ). AS is thought to regulate functional gene actions in two ways: by directly altering mRNA stability or by encoding distinct protein isoforms, which may influence physical interactions between the original protein and its associates [23] . The latter is frequently associated with AS that is regulated by environmental stress or temperature response [24] , [25] , [28] , [45] , [46] . Although we detected that FT2β / FT2α ratio was influenced by ambient temperature changes, the AS of FT2 may not be involved in temperature-mediated flowering control in B. distachyon , as increased ambient temperatures have limited influences on flowering signal induction in temperate grasses [43] . Interestingly, the FT2β / FT2α ratio was progressively reduced during development, indicating that FT2 AS is regulated by an endogenous cue rather than an external cue for fine-tuning plant flowering. FT2 AS may be modulated by some special splicing factors that abundance-, localization- or posttranslational modification-related changes as plant grow. Because miR156 and miR172 participate in the age-dependent regulation of flowering in diverse plants [12] , [13] , it will be interesting to explore whether alterations in FT2 growth-related AS in B. distachyon is controlled by these two miRNAs during flowering processes. FT2 and FT1 in B. distachyon are thought to have redundant roles on florigen activity because of their high amino-acid identities, similar temporal and spatial expression patterns, and same early flowering phenotype if overproduced. Thus it seems likely that FT2 and FT1 may have an analogous regulatory mechanism [14] , [15] . However, FT2 and FT1 are not regulated by identical schemes at the posttranscriptional level. First, their regulation by miR5200 is different. The base-pairing of miR5200 with the FT2 target site is not as perfect as that of FT1 , resulting in the cleavage of FT2 by miR5200 at a non-canonical miRNA cleavage site [14] . Second, FT2 ’s function is modulated by AS, which is altered during development to repress flowering in the early stage, while no FT1 AS events occur during the life cycle. Because both AS- and miRNA-mediated gene silencing are posttranscriptional gene regulatory mechanisms in eukaryotes, we propose that posttranscriptional modulation may be the major force for differentiating and fine-tuning different FT-like protein activities in Pooideae plants during evolution. In A. thaliana , BROTHER OF FT AND TFL1 (BFT), a member of the FT/TFL1 protein family, mediates the link between flowering and stress signaling [47] . BFT is expressed at low levels, irrespective of day length, but can be dramatically induced under highly saline conditions. BFT and FT have similar abilities to bind FD. Thus, when plants encounter salt stress, BFT causes delayed flowering by competing with FT for FD binding [47] . Similarly, TFL1 represses FT activity through its interactions with FD, which is involved in the prevention of flowering in immature meristems of A. thaliana , A. alpina and even apple trees [48] , [49] , [50] , [51] , [52] . In B. distachyon , although developmentally regulated FT2β also interferes with flowering initiation complex formation, its molecular mechanism is different from that of BFT in A. thaliana because FT2β does not bind FD. In a sense, FT2β functions as a competitor of FD, because both FT2β and FD can dimerize with FT2α . FT2β / FT2α ratio is high in young plants and this prevents the rapid progression towards flowering. If there was no FT2β generated at the vegetative stage, then the florigen activity conferred by either FT2α or FT1 would immediately exceed the threshold for the reproductive phase transition, which may lead to precocious flowering and detrimental effects on seed production. We found that full-length FT2 in B. distachyon can form homodimers and FT2-FT1 heterodimers. Similar findings that FT interacts with itself in A. thaliana suggest a possible biological relevance for the multimeric forms of FT proteins in plants [48] . Hence, further studies on when and where FT proteins form polymers in vivo will be important for determining their exact roles in accelerating flowering. Plants contain complex regulatory machineries to optimize the seasonal timing of flowering. Our present discovery of AS-mediated FT2 regulation in temperate grasses not only extends the manner of flowering control by FT but also reveals florigen control at both the transcriptional and posttranscriptional levels during the process of floral transition ( Fig. 7c ). In respect that multiple alternatively spliced forms of FT orthologous genes have been detected in Platanus acerifolia [53] , it will be interesting to determine whether the blocking flowering complex formation by splice variants is the same FT regulatory mechanism in trees. Plant materials and growth conditions B. distachyon used in this study were grown under LD conditions (16 h light/8 h dark) in growth chambers with temperatures of 22 °C during the day and 16 °C at night. For most experiments, the B. distachyon accession Bd21 was used. To minimize the crosstalk effects of photoperiod and vernalization on Bd21-3, seeds of transgenic and control plants were placed on moistened filter paper in Petri dishes and subjected to 4 °C cold treatment for 1 week before planting under the indicated conditions. Unless stated otherwise, all plant seedlings or leaves were harvested at Zeitgeber time 16 for use in the experiments. Constructs and plant transformation The FT2 ( FT2α and FT2β ) coding sequences and the miR172a backbone of the artificial miRNA were amplified from B. distachyon cDNA. FT2α , FT2β and artificial miRNAs constructs were all under the control of the maize ( Zea mays ) UBIQUITIN ( UBI ) promoter for overexpression in Bd21 or Bd21-3 plants. The sequences of the primers for B. distachyon FT2α , FT2β and artificial miRNA amplification, as well as for binary vector construction, are listed in Supplementary Table 1 . Transformation of B. distachyon was mediated by Agrobacterium tumefaciens strain AGL1 using compact embryogenic calli derived from immature embryos [54] . Independent transgenic lines were genotyped for T-DNA using HPT II -specific forward and reverse primers. The confirmed positive T 3 transgenic plants were used in flowering time determination and gene expression assays. Plant flowering time measurements The flowering times of the indicated plants were measured as the number of days from the date of planting in soil to the day when the first spike emerged. At least 10 plants of each transgenic line were recorded to calculate the average flowering time. Statistical significance was determined using Student’s t -test. RNA expression analysis Total RNA was isolated from at least three pooled B. distachyon plants using TRIzol reagent (Invitrogen). The total RNA sample was pretreated with RNase-free DNase I (Promega) prior to cDNA synthesis to remove DNA and then reverse transcribed by EasyScript reverse transcriptase (TransGen Biotech) using oligo (dT) primers. RT-PCR analyses of gene transcripts were essentially carried out as previously described [55] . qRT-PCR reactions were performed with SYBR Premix EX Taq (Takara) and run on an ABI 7,500 Fast system with the following procedure: 95 °C for 1 min, then 40 cycles of 95 °C for 10 s, 62 °C for 10 s, and 72 °C for 30 s, followed by a melting dissociation program. For the quantification of FT2α and FT2β transcripts, FT2α and FT2β cDNAs were cloned into pGADT7 vectors, and an absolute standard curve of each transcript was made using 10-fold serial dilutions from 10 −18 to 10 −23 mol μl −1 . The gene expression levels ( Fig. 5 and Supplementary Fig. 3 ) were calculated based on the ratio of absolute quantifications of FT2α and FT2β to the corresponding absolute value of UBC18 . For gene relative expression analysis, UBC18 mRNA was examined in parallel and used for data normalization, and the relative expression levels were calculated using the ΔΔCt method. All of the qRT-PCR analyses were performed at least in three independent biological replicates with three technical repetitions. For artificial miRNA detection, 2 μg total RNA was used for RNA gel blots. 32 P-end-labelled oligonucleotides complementary to the artificial miRNA sequences were used as probes. The sequences of the primers and small RNA blot probes are listed in Supplementary Table 1 . Yeast assays Yeast two-hybrid assays were conducted using the Matchmaker GAL4 Two-Hybrid System (Clontech). The PCR products of FT2α , FT2β , FT1 , FDL2 and diverse 14-3-3s from B. distachyon cDNA were independently cloned into the pGBKT7 and pGADT7 vectors. Transformation of AH109 cells was performed according to the general protocol. The transformed yeast cells were spread on the selective medium SD/-Leu/-Trp/-His/-Ade plus 2.5 mM 3-aminotriazole to determine the interactions. For the yeast three-hybrid assay, bait and prey were co-transformed with or without the competitor FT2β into yeast AH109 cells. The interaction strengths were quantified by a liquid β-Gal assay using chlorophenol red-β-D-galactopyranoside (CPRG) as substrates according to the Yeast Protocol Handbook (Clontech). Briefly, the yeast cells were broken open using several freeze/thaw cycles and mixed with CPRG buffer. When the colour of the sample turned to red, 3.0 mM ZnCl 2 was added to stop the reaction. The β-Gal units were calculated by the supernatant absorbance at 578 and 600 nm. BiFC assays To generate the constructs for the BiFC assays, full-length cDNA fragments of FT2α , FT2β , FT1 , FDL2 and GF14b were amplified and cloned into the pDONRZeo (Invitrogen) vector for fusion with the N-terminus of YFP or the C-terminus of CFP by LR reaction. The resulting plasmids were introduced into A. tumefaciens EHA105, which were then infiltrated into 4-week-old N. benthamiana leaves for transient expression. In brief, the A. tumefaciens strains were resuspended to OD600=0.8 in infiltration buffer (150 μM acetosyringone, 10 mM MgCl 2 and 10 mM MES). The resuspensions containing each BiFC construct as well as the p19 plasmid were mixed at 1:1:1 ratio and then infiltrated into leaves with a syringe. For the protein-binding competition assay, the A. tumefaciens harbouring the FT2β plasmid was co-infiltrated with an equal volume of the indicated construct. A. tumefaciens harbouring GUS in place of FT2β was infiltrated in parallel as a control. The tobacco leaves were imaged under Zeiss LSM 700 confocal microscope 3 days after infiltration. Excitation of YFP was performed using an argon laser line at 514 nm and red fluorescent protein (RFP) with 563 nm, while capture of YFP fluorescence was at 518–555 nm and RFP at 568–636 nm. Primers used to construct BiFC plasmids are shown in Supplementary Table 1 . Co-IP assays Full-length coding sequences of FT2α , FT2β and FDL2 were cloned into tagging plasmids under the control of Cauliflower Mosaic Virus 35S promoter. The 4-week-old N. benthamiana leaves were infiltrated with an A. tumefaciens strains harbouring FT2α-FLAG plus HA-FDL2 or FT2β-FLAG plus HA-FDL2. The infected leaves were collected 3 days after infiltration. Total protein was then extracted with IP buffer (50 mM Tris-HCl pH 7.5, 150 mM NaCl, 1 mM EDTA, 1% Triton X-100, 10% glycerol, 1 mM phenylmethyl sulfonyl fluoride, 1 mM NaVO 4 , 50 μM MG132 and 1 × protease inhibitor cocktail) and centrifuged three times at 16,000 g at 4 °C. The supernatant was incubated with Anti-Flag M2 Affinity Gel (Sigma, A2220) at 4 °C for 3 h with gentle shaking. After centrifugation at 600 g at 4 °C for 1 min, the agarose beads were washed five times with washing buffer (50 mM Tris-HCl pH 7.5, 150 mM NaCl, 1 mM EDTA, 0.1% Triton X-100). The precipitate was suspended, boiled in SDS loading buffer, separated by an SDS-PAGE and detected by anti-HA (Sigma, H6908, 1:5,000 dilution) or anti-FLAG antibody (Sigma, H7425, 1:3,000 dilution). The full scan picture of Co-IP assay results is shown in Supplementary Fig. 20 . Data availability The sequence of FT2β has been submitted to Genbank under accession code (KP637176). The authors declare that all other data that support the findings of this study are available in the manuscript and its Supplementary files or are available from the corresponding author upon request. How to cite this article: Qin, Z. et al . Regulation of FT splicing by an endogenous cue in temperate grasses. Nat. Commun. 8, 14320 doi: 10.1038/ncomms14320 (2017). Publisher’s note : Springer Nature remains neutral with regard to jurisdictional claims in published maps and institutional affiliations.